Fractal fronts of diffusion in microgravity Spatial scale invariance represents a remarkable feature of natural phenomena. A ubiquitous example is represented by miscible liquid phases undergoing diffusion. Theory and simulations predict that in the absence of gravity diffusion is characterized by long-ranged algebraic correlations. Experimental evidence of scale invariance generated by diffusion has been limited, because on Earth the development of long-range correlations is suppressed by gravity. Here we report experimental results obtained in microgravity during the flight of the FOTON M3 satellite. We find that during a diffusion process a dilute polymer solution exhibits scale-invariant concentration fluctuations with sizes ranging up to millimetres, and relaxation times as large as 1,000 s. The scale invariance is limited only by the finite size of the sample, in agreement with recent theoretical predictions. The presence of such fluctuations could possibly impact the growth of materials in microgravity. Spatial scale invariance is a notable feature of natural systems [1] , [2] , the most thoroughly investigated example being critical phenomena [3] , [4] . Scale invariance can also arise under rather generic conditions, even in the absence of critical behaviour [5] . An important model system in this respect is represented by miscible liquid phases undergoing diffusive remixing due to the random thermal motion of individual molecules. A long-standing, but incomplete, view is that it simply gives rise to a smooth mixing, unaccompanied by any significant perturbations of the diffusing fronts (surfaces of constant concentration). Theoretical models [6] , [7] , [8] and simulations [1] , [9] , [10] have suggested that the diffusing fronts are not smooth. Instead, they are predicted to exhibit a fractal structure with corrugations ranging in size from molecular to macroscopic, without the necessity of precisely tuning parameters to approach a critical point [5] . The development of truly long-range correlations in scale-invariant systems is suppressed by gravity, which limits the range to which fluctuations may grow. Extensive studies on critical phenomena have been performed under microgravity conditions to study the scale-invariant behaviour at macroscopic length scales [4] . In spite of the ubiquity of diffusive processes in nature, experimental investigation of long-range correlations in these systems has been limited, because of the fact that on Earth the development of such correlations at macroscopic length scales is severely affected by the presence of gravity. Depending on the direction of the diffusive flow with respect to gravity, the buoyancy force can either quench long-range concentration fluctuations [11] , [12] , [13] , [14] , [15] , [16] , [17] or amplify them [18] , [19] . Theoretical models [8] , [18] , [20] and simulations [1] , [9] , [10] of diffusive processes suggest that the absence of gravity should lead to the development of fractal fronts of diffusion where the largest length scale is limited only by the size of the sample, rather than by gravity. The presence of these fluctuations has a potential impact on the understanding of the growth of materials in the space, in particular for protein crystals [21] . Here we perform diffusion experiments in a polystyrene–toluene solution (MW=9,100 g mol −1 , average concentration 1.8 wt%) under microgravity conditions. The experiments were performed during the flight of FOTON M3 (ref. 22 ), a recoverable capsule inserted into orbit about 300 km above the surface of the Earth. The capsule is unmanned and fully automated, and this allows experiments to be performed in the presence of a low level of residual gravity (0.7 μg on average) at a relatively low budget [23] . The typical mission duration is of the order of 2 weeks. This allowed multiple sets of measurement cycles to be made, despite relaxation times as long as 1,000 s. By performing diffusion experiments under microgravity conditions, we have obtained unambiguous evidence that diffusion is accompanied by perturbations of the diffusion fronts with fractal structure, the largest perturbations involving regions with sizes of about 1 mm, and the slowest relaxation time being of the order of 1,000 s. The only limitation to the scale-invariant behaviour of the perturbations is due to the finite thickness of the sample, which imposes an upper limit on the amplitude of fluctuations. Our results are in good agreement with theoretical predictions for the dependence of the mean-squared amplitude of the fluctuations on wave vector obtained by using linearized Boussinesq hydrodynamics [8] , [18] . We also show that the relaxation times of the perturbations are fully compatible with diffusion, even at wave vectors where the finite size of the container significantly affects the mean-squared amplitude of the fluctuations. Although this result was not predicted a priori , we have extended the one-mode Galerkin model [8] , [18] to include dynamics, and find predictions numerically consistent with the experimental data. Beyond their fundamental interest, our results are relevant for understanding the results of experiments involving diffusion performed in microgravity to exploit the absence of convection. Although convection is assumed to be absent in such experiments, the large amplitude and long-lived perturbations reported in this work should be taken into account to achieve a deeper understanding of results obtained in the microgravity environment. Experimental diagnostics Performing a classical free-diffusion experiment necessitates bringing two miscible liquid phases into contact while avoiding accidental perturbation of the interface [13] , [17] . An alternative, robust approach suitable for microgravity experiment is to use the Soret effect [24] . Imposition of a steady temperature difference Δ T across the polystyrene–toluene mixture induced a concentration difference Δ c , with the polymer chains migrating towards the colder side. The resulting steady-state concentration profile is governed by ∇ c =− S T c (1− c ) ∇ T . Here S T =6.49×10 −2 K −1 is the Soret coefficient, and c is the concentration. The magnitude of the concentration difference can be readily altered, and the experiment repeated as desired. The thermal-gradient cell was a flight-engineered version of a prototype used for ground-based tests [25] , and was similar to designs developed previously [12] , [13] . The sample was a 25 mm diameter by 1.00-mm-thick layer of polymer solution confined between two parallel, 12-mm thick, sapphire windows that were temperature controlled to better than ±0.01 K. The use of sapphire windows allowed the application of a relatively uniform temperature difference, whereas permitting optical access to the sample in a direction parallel to the imposed gradient. The sample was illuminated with collimated, 680 nm wavelength, light from a super-luminous light emitting diode (LED) coupled to a mono-mode optical fibre. Interference between the beam and the light scattered by the diffusing fronts resulted in small, but measurable variations of the intensity in the images collected by a charge-coupled device with 1,024×1,024 square pixels. The central 512×512 portion of differences of succeeding images were Fourier decomposed to reveal the mean-squared amplitude of concentration fluctuations versus the scattering wave vector q . A measurement cycle involved an initial equilibration phase at a uniform temperature of 30.0 °C for 260 min. Towards the end of this phase, a set of 539 reference images was acquired to characterize the optical background and the camera noise. This phase was followed by the rapid imposition of a temperature difference across the sample, which started the diffusion process. The temperature differences utilized were 4.35, 8.70 and 17.40 K. The time required for the formation of a linear temperature profile was about 100 s. In contrast, the time to create a steady-state concentration profile ( τ o = h 2 /( π 2 D )) was about 500 s; here D =1.97×10 −6 cm 2 s −1 is the diffusion coefficient, and h =1.00 mm the sample thickness. The development of nonequilibrium concentration fluctuations on Earth and in space We used the quantitative shadowgraph method [26] , [27] , [28] , [29] to measure the scattering of light from the diffusing fronts, which would be parallel planes and scatter no light in the absence of fluctuations. This method has a high degree of immunity to stray elastically scattered light, and it does not require sensitive alignment of optical components, making it an excellent technique for microgravity. A drawback is that it is characterized by an oscillatory transfer function T ( q ), which requires an accurate calibration. As a concentration gradient was created, millimetre-scale concentration fluctuations became discernable. 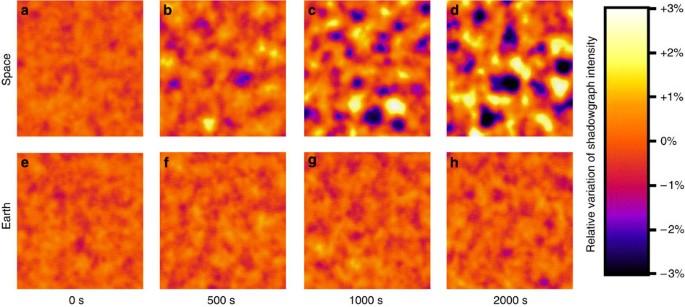Figure 1: Development of nonequilibrium fluctuations during diffusion processes occurring on Earth and in space. False-colour shadowgraph images of nonequilibrium fluctuations in microgravity (a–d) and on Earth (e–h) in a 1.00-mm-thick sample of polystyrene in toluene. Images were taken 0, 400, 800, and 1,600 s (left to right) after the imposition of a 17.40 K temperature difference. The side of each image corresponds to 5 mm. Colours map the deviation of the intensity of shadowgraph images with respect to the time-averaged intensity. This is shown by the upper row of images in Figure 1 , which displays a sequence of false-colour shadowgraph images obtained in microgravity at different times after the imposition of a 17.40 K temperature difference. For comparison, the lower row shows images acquired on Earth under the same conditions. In the experiment carried out on Earth, the sample was heated from above, and thus was completely stable against convective motion. The sequence shown in Figure 1 is also provided as a movie (see Supplementary Movie 1 ), in which the dynamics corresponding to the fluctuations is apparent. The same experiment is performed simultaneously in space (left) and on ground (right). The sample was initially isothermal, a configuration in which the concentration of polymer is uniform. A temperature difference of 17.4 °C was then rapidly applied across the sample, as indicated in the video (gradient on). The thermophobic polymer chains migrate towards the cold plate, and this thermophoretic flux is opposed by a diffusive flux that increases until it reaches steady state when the concentration difference Δ c is fully established. Once a significant concentration difference has developed, concentration fluctuations become visible both in space and on Earth, with those in space clearly being much larger, both in physical extent and amplitude. In addition, one can see that the long-ranged fluctuations observed in space evolve over much longer timescales than do the shorter-ranged, smaller amplitude fluctuations observed on the Earth. Figure 1: Development of nonequilibrium fluctuations during diffusion processes occurring on Earth and in space. False-colour shadowgraph images of nonequilibrium fluctuations in microgravity ( a – d ) and on Earth ( e – h ) in a 1.00-mm-thick sample of polystyrene in toluene. Images were taken 0, 400, 800, and 1,600 s (left to right) after the imposition of a 17.40 K temperature difference. The side of each image corresponds to 5 mm. Colours map the deviation of the intensity of shadowgraph images with respect to the time-averaged intensity. Full size image Mean-squared amplitude of the nonequilibrium concentration fluctuations The temperature difference was held constant for 42 h, and images of the fluctuations were recorded every 10 s. The series of about 15,000 images thus obtained allowed us to perform a quantitative analysis of the statistical properties of the concentration fluctuations. The analysis relies on the decomposition of the shadowgraph images into Fourier modes of wave vector q , to determine the mean-squared amplitude of concentration fluctuations S c ( q ). Although S c ( q ) is a static quantity, its determination was best achieved by performing a dynamic analysis using sequences of shadowgraph images. This is due to the fact that shadowgraph images obtained from a polymer solution in the presence of a temperature difference include additional contributions from equilibrium temperature and concentration fluctuations, as well as from nonequilibrium temperature fluctuations. Only the latter are large enough to contribute detectable signal, but they occur on time scales that are sufficiently fast that their contribution is uncorrelated between images. Consequently, their contribution appears in the form of an additive background and can be removed. Other sources of uncorrelated contributions to the images include shot noise associated with the photon-detection process and noise from the camera electronics, both of which also contribute only to the additive background. By analysing the temporal properties of sequences of shadowgraph images, we were able to isolate the portion attributable to the concentration fluctuations. The division of this portion of the signal by the instrumental transfer function T ( q ) allowed determination of the mean-squared amplitude S c ( q ) of concentration fluctuations to within an arbitrary factor. 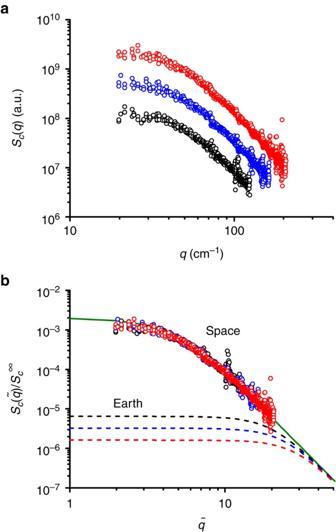Figure 2: Mean-squared amplitude of nonequilibrium concentration fluctuations in microgravity. (a) Experimental results obtained in microgravity in the presence of temperature differences of 4.35 K (black circles), 8.70 K (blue circles) and 17.40 K (red circles). (b) Comparison of the experimental results with the theoretical predictions8,18. The solid line represents the theoretical prediction for microgravity. The dashed lines are the theoretical predictions for the power spectra of the nonequilibrium concentration fluctuations on the Earth. In microgravity, the data scale onto a single universal curve, whereas on the Earth no such scaling occurs. The results obtained from image sequences in the presence of temperature differences of 4.35, 8.70 and 17.40 K are shown in Figure 2a . Figure 2: Mean-squared amplitude of nonequilibrium concentration fluctuations in microgravity. ( a ) Experimental results obtained in microgravity in the presence of temperature differences of 4.35 K (black circles), 8.70 K (blue circles) and 17.40 K (red circles). ( b ) Comparison of the experimental results with the theoretical predictions [8] , [18] . The solid line represents the theoretical prediction for microgravity. The dashed lines are the theoretical predictions for the power spectra of the nonequilibrium concentration fluctuations on the Earth. In microgravity, the data scale onto a single universal curve, whereas on the Earth no such scaling occurs. Full size image The data for large q are consistent with a power law behaviour S c ( q ) ∝ q −4 , which characterizes scale-invariant fluctuations on fractal diffusing fronts. At sufficiently small q , even in the absence of gravity, the divergence saturates due to the boundaries, which limit the development of fluctuations with wave vectors below about q X ≈ π / h ≈31.4 cm −1 for our sample. Figure 2b shows that all three data sets collapse onto a single master curve when scaled in the manner described below. Relaxation times of the perturbations Image sequences (see Supplementary Movie 1 ) show the continuous temporal and spatial evolution of the fluctuations. The dynamic analysis allowed us to measure the relaxation time τ c ( q ) of the perturbations. 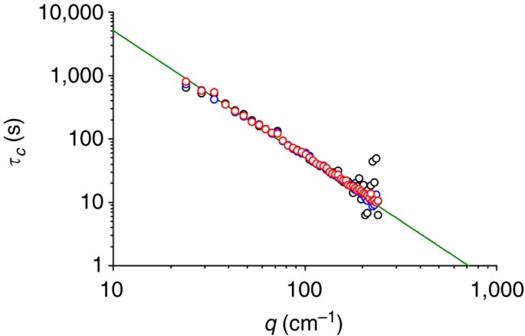Figure 3: Relaxation time of non-equilibrium concentration fluctuations as a function of wave vector. The black data correspond to a temperature difference of 4.35 K, the blue data to 8.70 K and the red ones to 17.40 K. The solid line represents the diffusive timeτc(q)=1/(Dq2) as estimated from literature data for the diffusion coefficient. The relaxation times obtained in this manner are shown in Figure 3 as a function of wave vector. Figure 3: Relaxation time of non-equilibrium concentration fluctuations as a function of wave vector. The black data correspond to a temperature difference of 4.35 K, the blue data to 8.70 K and the red ones to 17.40 K. The solid line represents the diffusive time τ c ( q )=1/( Dq 2 ) as estimated from literature data for the diffusion coefficient. Full size image The black, blue and red data correspond to temperature differences of 4.35, 8.70 and 17.40 K, respectively. The solid line represents the diffusive relaxation time τ c ( q )=1/( Dq 2 ), obtained independently by using the literature value for the diffusion coefficient. The measured relaxation times are fully compatible with mass diffusion, and this provides a straightforward demonstration that the concentration fluctuations observed in microgravity are an intrinsic feature of diffusion. Interestingly, in the observed wave vector range the relaxation times do not seem to be affected by the finite thickness of the sample, despite the measurable effects on S c ( q ). We speculate that this is due to the fact that the boundaries cannot transfer mass, only heat. Therefore, concentration fluctuations can relax back to equilibrium only through diffusion. In the absence of gravity, and with the radius of gyration of the polymer chains much larger than the size of solvent molecules, a theoretical model [8] , [18] based on a single-mode Galerkin approximation predicts that the mean-squared amplitude of fluctuations should scale onto a universal curve independent of mixture properties or applied concentration difference. Here Λ≈4.73, B =Λ tanh (Λ/2) [2Λ tanh (Λ/2)−4]≈24.6, and is the dimensionless wave vector. The asymptotic value at large wave vectors used to normalize the data is defined as Thus, the theoretical master curve scales as q̃ −4 at large wave vectors and saturates to a constant value at small wave vectors. The asymptotic value used to normalize the experimental data was determined by fitting the data at q̃ > 8 with a power-law function This normalization scheme allows a quantitative comparison between the predictions and the experimental results. Figure 2b shows the data plotted with the theoretical prediction, in the absence of adjustable parameters. The experimental results provide a straightforward confirmation of the scale invariance of the fluctuations up to wavelengths comparable to the sample thickness. Above this length scale, the results confirm that the scale invariance of the fronts of diffusion is frustrated by the finite size of the container, as predicted by theory [18] and by recent two-dimensional simulations [10] . The dashed curves in Figure 2b show the theoretical predictions for the mean-squared amplitude of fluctuations on the Earth. Clearly, gravity would give rise to a non-universal behaviour at low q , whereas in the microgravity the only relevant parameter is sample thickness. Our observation of diffusive relaxation times throughout the entire range of explored wave vectors represents a simple and remarkable result. Although explicit analytic results for the dynamics have not been published yet, we have extended the one-mode Galerkin model [8] , [18] to achieve a numerical calculation of the relaxation times. We find that, although the decay is not predicted to be exactly diffusive, it is very nearly so. The limitations involved in the approximate Galerkin model can be overcome by using an exact model to predict the behaviour of the relaxation times as a function of wave vector in the presence of finite size effects [20] . However, although such an exact model allows one to obtain refined quantitative estimates, analytic expressions and systematic numerical estimates of the relaxation times are not yet available, and we hope that our experimental results will stimulate further theoretical work. One implication of this experiment is that when dealing with processes controlled by diffusion, microgravity is not necessarily the simple quiet environment that is usually imagined. Microgravity conditions are routinely exploited to investigate the diffusive growth of materials, because of the absence of convective motion. Studies of such processes have involved a detailed analysis of the advantages related to the absence of convection, but they have not yet considered the possible effects of long-ranged, extremely long-duration, nonequilibrium fluctuations enhanced by the absence of gravity. A notable example of a system in which fluctuations similar to those reported here could have a role is the crystallization of proteins in microgravity [21] , wherein the crystallization process occurs because of the diffusive transport of proteins towards the growing crystal, which is surely accompanied by such fluctuations. Determination of wave vectors The discrete Fourier transform of an image of side length W provides data points corresponding to two-dimensional wave vectors having components of the form ± pq Min , p =0,1,2... with q Min =2 π / W . To determine the value of q Min in cm −1 , it is necessary to relate pixel size to physical dimension. We used the known Fresnel interference pattern of the circular boundary of the sample to achieve this calibration to an accuracy of about 1%, with the result being q Min =4.80 cm −1 . Calibration of the optical system Quantitative shadowgraphy is a simple, yet powerful, method of detecting weak phase perturbations by measuring intensity modulations of the transmitted beam a distance z from the sample. The intensity modulations result from interference between the main beam and light diffracted by the perturbations. The method is characterized by a damped oscillatory transfer function, which may be written as T ( q )= A ( q ) sin 2 [ q 2 z /(2 k 0 )]+ C ( q ), in which the envelopes of the minima and maxima are equal to C ( q ) and A ( q )+ C ( q ), respectively. Both A ( q ) and C ( q ) decay with increasing wave vector because of a variety of instrumental effects. Calibrating the optical system means basically to determine the functions A ( q ) and C ( q ). Suspensions of small colloidal particles are ideal for shadowgraph calibration, as they also are for conventional light scattering. We selected polystyrene latex spheres of diameter 2.0 μm suspended in isopropyl alcohol, as they provide a large signal, and are small enough to scatter light uniformly for the wave vector range of interest. To carry out the calibration, 320 images were taken with the cell filled with filtered isopropyl alcohol, to determine a background signal S B ( q ). The cell was then filled with the colloidal suspension and 3,500 images were taken. Between each image, the sample was stirred using an automatic piston, to ensure statistically independent images. After subtracting S B ( q ), the signal from the spheres is given by S Sp ( q )= A ( q ) sin 2 [ q 2 z /(2 k 0 )+ ϕ Sp ]+ C ( q ), where ϕ Sp is an additional phase delay that accounts for the non-vanishing optical thickness of the 2 μm spheres in isopropyl alcohol [30] . We found the phase delay to be 1.78 radians, in very good agreement with Mie theory [31] . The functions A ( q ) and C ( q ) were determined by fitting the data for S Sp ( q ), and this in turn allowed us to determine the instrumental transfer function T ( q ). Measurement cycles During the flight, six scientific measurement cycles were performed. Each cycle was composed of the phases detailed in the following: (A) stabilization of the sample and electronics at 30 °C (170 min). (B) acquisition of 539 background images in the absence of diffusion (90 min). (C) Imposition of a temperature difference and acquisition of 199 images showing the development of concentration fluctuations (33 min). (D) Acquisition of 15,277 images of nonequilibrium fluctuations in the presence of a steady gradient (2,533 min). (E) Removal of temperature difference and acquisition of 199 images. Dynamic processing The dynamic analysis involved the processing of sequences of 5,000 images to calculate the structure function D I ( q , τ )=〈| I ( q , t )− I ( q , t + τ )| 2 〉, at 65,600 different wave vectors. For an ergodic stationary process, such as we are studying, the structure function is related to the more familiar correlation function G I ( q , τ ), by D I ( q , τ )=2( G I ( q , 0)− G I ( q , τ )), but has the advantage of being less sensitive to slowly changing experimental effects [32] . After averaging over wave vectors of the same magnitude q , the structure function was fitted using a single exponential where S c ( q ), τ c ( q ) and B ( q ) were adjusted in fitting. Here T ( q ) is the instrumental transfer function and B ( q ) is a background due to nonequilibrium temperature fluctuations (which are sufficiently rapid that their contributions are uncorrelated between images) and detector noise. For all wave vectors analysed, a single exponential fit well, ruling out contributions other than those coming from concentration fluctuations. The instrumental transfer function T ( q ) was determined on the Earth by using the procedure outlined above in the calibration section. Processing of Supplementary Movie 1 The sequence is composed of square images of size 350 pixels (corresponding to ∼ 9 mm) obtained near the centre of the 25-mm diameter sample. Images were recorded every 10 s, and at 25 frames per sec are being shown at 250 times the actual speed. The arbitrary false-colour scale was derived from the 10-bit data images produced by the charge-coupled device camera. After subtraction of a time-independent background image, images were low-pass filtered with a Gaussian to reduce high-spatial frequencies. Such filtering was not applied to the dynamic processing of the data described above. How to cite this article: Vailati, A. et al . Fractal fronts of diffusion in microgravity. Nat. Commun. 2:290 doi: 10.1038/ncomms1290 (2011).